Chiral superfluidity withp-wave symmetry from an interactings-wave atomic Fermi gas Chiral p -wave superfluids are fascinating topological quantum states of matter that have been found in the liquid 3 He-A phase and arguably in the electronic Sr 2 RuO 4 superconductor. They are fundamentally related to the fractional 5/2 quantum Hall state, which supports fractional exotic excitations. Past studies show that they require spin-triplet pairing of fermions by p -wave interaction. Here we report that a p -wave chiral superfluid state can arise from spin-singlet pairing for an s -wave interacting atomic Fermi gas in an optical lattice. This p -wave state is conceptually distinct from all previous conventional p -wave states as it is for the centre-of-mass motion, instead of the relative motion. It leads to spontaneous generation of angular momentum, finite Chern numbers and topologically protected chiral fermionic zero modes bounded to domain walls, all occuring at a higher critical temperature in relative scales. Signature quantities are predicted for the cold atom experimental condition. Topological superconductors, like the type of p x + ip y -wave pairing studied in the liquid 3 He (ref. 1 ) and strontium ruthenates [2] , are among the most desirable unconventional many-body states in condensed matter physics [3] . In two dimensions (2Ds), their topological properties are fundamentally linked to a class of fractional quantum Hall states of non-Abelian statistics [4] . Studies of vortices in such materials point to fascinating braiding statistics and applications in topological quantum computing. The fate of topological superconductivity in 2D electronic matter remains, however, debatable. In the field of ultracold atoms, this phase was predicted to appear near the p -wave Feshbach resonance in Fermi gases [5] . However, the life time of such systems is severely limited by the three-body collisions, and achieving superfluidity in the resonance regime was found experimentally challenging [6] . Creating the equivalent of p -wave interactions using spin-orbit coupling or dipolar interactions provides a different interesting approach [7] , [8] , for which future experimental breakthroughs are desired to suppress heating or ultracold chemical reactions. Another approach proposed to get around [9] is to hybridize materials of topological and superconducting properties. This approach nevertheless requires advanced material engineering. After all, the search for chiral p -wave superconductivity in 2Ds has stood largely open for both electronic and atomic matter systems. Here we report the discovery of a new mechanism to achieve chiral topological superfluidity. We shall introduce this with a specific model of cold fermionic atoms in an optical lattice, to be described below. The key idea is a centre-of-mass p -wave superconducting pairing. Unlike the past models that require a p -wave two-body interaction or induced ones [10] , [11] , [12] , [13] , [14] , [15] , [16] , [17] , [18] , the present pairing mechanism departs from the conventional reliance on p -wave pairing in relative motion. Here the pairing of fermions takes place between s and p orbitals, which have even and odd parity, respectively. Recently, the research of higher orbital bands in optical lattices has evolved rapidly [19] , where the orbital degrees of freedom are found to play a crucial role as in solid-state materials. From the early experimental attempt [20] to the breakthrough observation [21] of long-lived p -band bosonic atoms in a checkerboard lattice, a growing evidence points to an exotic p x + ip y orbital Bose–Einstein condensate [19] . For fermions studied in this work, the decay from higher to lower bands is prevented by Pauli blocking, and the fermionic p -band system is even more robust than the bosonic counterpart. Concerning p -band fermions with attractive interaction, superfluid states similar to the type of Fulde–Ferrell–Larkin–Ovchinnikov were found in the theoretical studies of pairing within the p -bands [22] and that between the s -band and a single p -band [23] . As we shall show with the model below, pairing fermions from the orbitals of different angular momenta can lead to other unexpected results. Effective model Let us consider an attractive s -wave-interacting Fermi gas composed of two hyperfine states, to be referred to as spin ↑ and ↓, loaded in a spin-dependent 2D optical lattice shown in Fig. 1a . The spin dependence of the lattice is motivated by various theoretical designs [24] , [25] and most importantly the recent experimental demonstration of it with bosons [26] , [27] . Further, let the gas be tuned with a population imbalance between the two spin species by the techniques developed in the recent experimental advances [28] , [29] , [30] . A key condition that we propose here is to tune the population imbalance (or equivalently the chemical potential difference) sufficiently large such that the spin ↑ and ↓ Fermi levels reside in the s and p orbital bands, respectively. The rotation symmetry ( C 4 ) of the lattice dictates that the two p orbital bands, p x and p y , are degenerated at the high symmetry points in the momentum space. Later on we shall see that this symmetry and hence degeneracy are necessary for the p x + ip y -wave paired superfluidity. Technically speaking, the Bravais lattices for the spin up and down fermions are 45° rotated from each other. 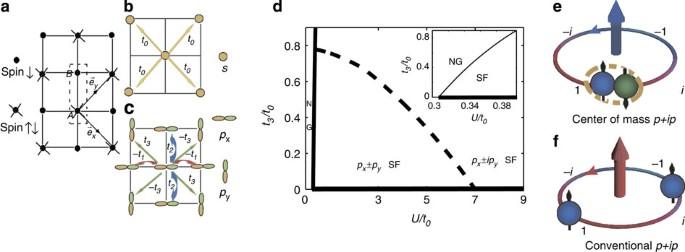Figure 1: Optical lattice system and zero-temperature phase diagram. (a) Schematic picture of a 2D spin-dependent optical lattice, where the spin up (sorbital band) and down (porbital band) component lying within different geometry lattice potential, respectively. HereAandBstand for two different sites in one unit cell,andare the primitive unit vectors. (bandc) Schematic views illustrate tunnellingt0,t1,t2andt3of fermions prepared in thesandporbitals, respectively. (d) Zero-temperature phase diagram whent1/t0=8,t2/t0=2—The solid line illustrates the phase transition from normal gas (NG) to superfluid state (SF). WhenU/t0<7, the critical value oft3/t0as shown by the dash line, beyond this threshold a phase transition frompx±pytopx±ipysuperfluid state occurs. WhenU/t0≥7,px±ipysuperfluid state is the ground state with non-zerot3. The thick solid line stands for a two-component superfluid state. (eandf) Pictorially illustrate the distinction between centre-of-mass and conventionalp+ippairings. Here, the character ofp+ippairing states is demonstrated by the phase of the superconducting gap labelled by the colour of the torus. Ine, the Cooper pair is a spin-singlet pair composed of two spin species fermions and has finite centre-of-mass orbital angular momentum, whereas infit is a conventional spin-triplet pair formed by single species fermions and has conventional relative motion angular momentum. Figure 1: Optical lattice system and zero-temperature phase diagram. ( a ) Schematic picture of a 2D spin-dependent optical lattice, where the spin up ( s orbital band) and down ( p orbital band) component lying within different geometry lattice potential, respectively. Here A and B stand for two different sites in one unit cell, and are the primitive unit vectors. ( b and c ) Schematic views illustrate tunnelling t 0 , t 1 , t 2 and t 3 of fermions prepared in the s and p orbitals, respectively. ( d ) Zero-temperature phase diagram when t 1 / t 0 =8, t 2 / t 0 =2—The solid line illustrates the phase transition from normal gas (NG) to superfluid state (SF). When U / t 0 <7, the critical value of t 3 / t 0 as shown by the dash line, beyond this threshold a phase transition from p x ± p y to p x ± ip y superfluid state occurs. When U / t 0 ≥7, p x ± ip y superfluid state is the ground state with non-zero t 3 . The thick solid line stands for a two-component superfluid state. ( e and f ) Pictorially illustrate the distinction between centre-of-mass and conventional p + ip pairings. Here, the character of p + ip pairing states is demonstrated by the phase of the superconducting gap labelled by the colour of the torus. In e , the Cooper pair is a spin-singlet pair composed of two spin species fermions and has finite centre-of-mass orbital angular momentum, whereas in f it is a conventional spin-triplet pair formed by single species fermions and has conventional relative motion angular momentum. Full size image A system of fermionic atoms, say 6 Li, loaded into an optical lattice ( Fig. 1a ) in the tight binding regime is described by a multi-orbital Fermi Hubbard model where H 0 describes tunnelling pictorially represented in Fig. 1b,c (the expression for H 0 is standard and is given in Supplementary Note 1 ) and H int is the Hubbard interaction, Here is a fermionic annihilation operator for the localized ν ( s , p x or p y ) orbital on A sites and the corresponding annihilation operator on the B sites is denoted as with R labels the lattice site. The interactions between s and p orbitals originate from interactions between two hyperfine states, which are tunable by the s -wave Feshbach resonance in ultracold atomic gases. We focus on the case with attractive interaction where superconducting pairing is energetically favourable. Although the annihilation operators do not appear in the interaction H int , they play important roles in the tunnelling Hamiltonian H 0 by determining the orientation of Fermi surfaces. With spin ↓ fermions residing on both A and B sites, and spin ↑ once on A sites only, Fermi surfaces of the s -band for spin ↑ and the p -band for spin ↓ are approximately two squares right on top of each other. Such a momentum-space geometry leads to nearly perfect Fermi surface nesting, which is the key to the p -wave superconducting pairing between s and p orbitals at weak interaction. The system, as described by the Hamiltonian in equation (1), exhibits lattice rotation C 4 and reflection symmetries. For the reflection in the horizontal and vertical direction (see Fig. 1a ), the fermionic operators transform as and , respectively. Under the lattice rotation, . These symmetries, reflection symmetries in particular, play an essential role in the following theory. Ginzburg–Landau theory From the analysis of Cooper’s problem (see Supplementary Note 2 and Supplementary Fig. 1 ), we conclude that condensation of Cooper pairs at Q =( π / a , π / a ) is most energetically favourable in the ground state, where a is the lattice constant. This peculiar momentum selection for Cooper pairs is related to the Fermi surface nesting at half-filling. Then, it is convenient to introduce two slowly varying bosonic fields Δ x ( x ) and Δ y ( x ), which represent Cooper pairs and in the low-energy limit, respectively, with x a coarse grained coordinate for the lattice labelling R . The pairing fields Δ x ( x ) and Δ y ( x ) are parity odd and transform as Δ x ( x , y )→ −Δ x (− y ,− x ), Δ y ( x , y )→Δ y (− y ,− x ) and Δ x ( x , y )→Δ x ( y , x ), Δ y ( x , y )→−Δ y ( y , x ) under reflection in the horizontal and vertical directions (see Fig. 1a ), respectively. The symmetry of the pairing fields plays a crucial role in determining the form of the free energy, to be demonstrated in the following. A two-flavour Ginzburg–Landau free energy respecting all the symmetries is given as follows with and f Gaussian = K (|∂ x Δ x | 2 +|∂ y Δ y | 2 +|∂ x Δ y | 2 +|∂ y Δ x | 2 ). Here r , g 1 , g 2 , g 3 and K are phenomenological coefficients to be related to the Hamiltonian (equation (1)) by microscopic calculations. This free energy generalizes the theory of two-gap superconductivity as proposed in the context of transition metals [31] . We have neglected temporal fluctuations of Cooper pair fields and such a treatment is valid at non-zero temperature away from quantum critical regime. In this theory, we want to emphasize two key points owing to the reflection symmetries: first, Δ x and Δ y are decoupled at quadratic level; second, linear derivatives such as are prohibited. The absence of linear derivatives makes modulations in Δ x \ y suppressed, and condensation of Cooper pairs at ( π / a , π / a ) is expected to be stable against weak perturbations such as having small t 2 ( Fig. 1c ) or slightly doping away from half-filling. For finite t 2 and t 3 ( Fig. 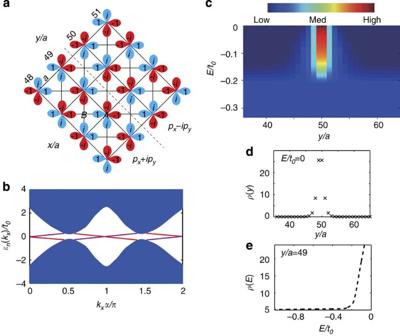Figure 2: Topological domain wall defect. (a) Schematic picture of a lattice system in the presence of a domain wall. (b) Energy spectrum of the system with a domain wall defect, whent1/t0=8,t2/t0=2,t3/t0=0.1 andU/t0=9. The purple and red branches correspond to the modes at the domain wall and the edge of the lattice, respectively. (c–e) The local density of states (LDOS) defined in the main text. The peak of LDOS located at domain wall is shown by red colour incand further shown withE/t0=0 andy/a=49 indande, respectively. The LDOS is in units of 1/at0. 1c ), the stability (that is, K >0 in equation (3)) is confirmed in our numerics (see Supplementary Note 3 and Supplementary Figure 2 ). The rotation symmetry plays another key role. For example, it protects the degeneracy of the two components Δ x and Δ y , that is, the splitting terms such as |Δ x | 2 −|Δ y | 2 are not allowed in the free energy. In short, the point group D 4 symmetry protects the form of the free energy in equation (3). Here we point out that the preserved space lattice rotation symmetry makes our model different from the spin-orbit-coupled systems, where such symmetry is absent. With the phenomenological coefficients r and g 3 obtained from integrating out fermions (see Supplementary Fig. 2 ), we find a phase diagram shown in Fig. 1d . With moderate attraction U <7 t 0 , a first-order phase transition from the p x ± p y to p x ± ip y phase occurs when the diagonal hopping t 3 is above some critical value. Surprisingly, when the attraction is strong enough U >7 t 0 , we find that even infinitesimal t 3 makes the p x ± ip y favourable, opening a wide window for this non-trivial state. When t 3 =0, the system has U (1) × U (1) symmetry, which means no phase coherence between the two components Δ x and Δ y . We also find that the superconducting gaps Δ x and Δ y have anisotropy in momentum space (see Supplementary Note 5 and Supplementary Fig. 4 ). Here we emphasize the crucial role of t 3 in determining the relative phase between Cooper pairs Δ x and Δ y . As it mixes the p x and p y orbitals, the particle numbers of these two orbitals are no longer separately conserved, and will consequently lock the relative phase between these two pairing fields. For large t 3 , the p x ± ip y state mostly minimizes the free energy and becomes energetically favourable. Surprisingly, this p x ± ip y phase is found to occupy a large region in the phase diagram ( Fig. 1d ). In the strong interaction regime, Cooper pairs behave like tightly bound repulsive molecules and the energetic selection of the p x ± ip y phase can be understood from an analogue of Hund’s rule for p -orbital bosons [32] , where maximizing the angular momentum generically saves the interaction energy cost. The p -wave superfluidity proposed here refers to a centre-of-mass p -wave pairing state. The distinction of such pairing from the conventional spin-triplet pairing p x + ip y states is illustrated in Fig. 1e,f . To further distinguish this state from the conventional relative p -wave pairing that usually involves two different sites (for example, pairs between spinless fermions) owing to the fermionic statistics, we consider a general pairing form Φ COM ( x , x′ ), which represents the Cooper pair between parity even and odd orbitals (that is, s and p orbitals) from any two sites. Under parity transformation, the pairing transforms as Φ COM ( x , x′ )→−Φ COM (− x ,− x′ ), rather than Φ COM ( x , x′ )→−Φ COM ( x′ , x ), which distinguishes the centre-of-mass from the conventional relative p -wave pairing. A remarkable feature immediately borne out of this pairing mechanism is the centre-of-mass p -wave superfluidity arises directly from a purely s -wave two-body interaction, requiring neither engineered p -wave interactions nor induced effective ones. This leads to a significantly improved transition temperature, which is confirmed by our study of the finite temperature phase transitions for the model Hamiltonian (equation (1); see Supplementary Note 4 and Supplementary Figure 3 ). For example, taking a typical density of the 40 K gas [33] , [34] and the potential depths of the optical lattice to be V s / E R =3 and V p /2 E R =5 for s and p orbitals (see the lattice potentials in Methods), respectively, we estimate the Kosterlitz–Thouless transition temperature can reach around 100 nK or higher, being within the experimental temperature scope [35] . Gapless chiral fermions We now show that the p x ± ip y superfluid state possesses important measurable signatures because of the broken time reversal Z 2 symmetry, which belongs to the Ising universality class. Following the standard procedure, our calculation finds that the state is topologically nontrivial by a non-zero Chern number, which is 1 and −1 for the p x + ip y and p x − ip y state, respectively. The topological properties are manifested in the existence of gapless chiral fermions, emergent on a domain wall connecting topologically distinct regions. In experiments, Ising domains of p x + ip y and p x − ip y are expected to spontaneously form as have been observed in the recent cold atom experiment studying ferromagnetic transitions [36] . In the following, we show that a domain wall defect carrying gapless fermions as bounded surface states is experimentally accessible. Considering a lattice geometry in the presence of a domain wall decorated superconducting background as in Fig. 2a , the mean-field Hamiltonian is given by Figure 2: Topological domain wall defect. ( a ) Schematic picture of a lattice system in the presence of a domain wall. ( b ) Energy spectrum of the system with a domain wall defect, when t 1 / t 0 =8, t 2 / t 0 =2, t 3 / t 0 =0.1 and U / t 0 =9. The purple and red branches correspond to the modes at the domain wall and the edge of the lattice, respectively. ( c – e ) The local density of states (LDOS) defined in the main text. The peak of LDOS located at domain wall is shown by red colour in c and further shown with E / t 0 =0 and y / a =49 in d and e , respectively. The LDOS is in units of 1/ at 0 . Full size image Here we emphasize that the centre-of-mass p -wave superfluidity, as described in equation (4), exhibits an unbroken spin U (1) symmetry under the transformation and . Such an unbroken continuous symmetry is absent in the conventional relative p -wave pairing state for either spinless or spin-orbit-coupled fermion systems. The energy spectrum of fermionic excitations is obtained by diagonalizing equation (4). With the periodical boundary condition chosen in the x direction ( Fig. 2a ), the momentum k x is a good quantum number and the energy spectra in Fig. 2b is thus labelled by k x . For the same reason as in quantum Hall insulators, the number of gapless chiral modes moving along the interface is topologically determined by the difference of the Chern numbers in regions on either side of the interface [37] ; in this case, |Δ C |=2. This conclusion is confirmed in our numerics. As shown in Fig. 2b , we find four gapless chiral modes, with two localized on the domain wall (purple colour) and the other two on the outer edges of the lattice (red colour). From their spectra ε n ( k x ), the two chiral modes on the domain wall have positive group velocities, which lead to anomalous mass flow along the domain wall [38] . Experimental signatures Several different methods can be used to observe our proposed chiral p -wave superfluidity experimentally. For instance, one of the direct experimental evidence for this topological superfluids, as in quantum Hall insulators, is the existence of the gapless chiral edge states. The domain wall supporting gapless chiral fermions between two Ising domains p x + ip y and p x − ip y can spontaneously form in atomic gases in a trap. These gapless fermionic states lead to signatures in local density of states (LDOS), which can be measured by radio-frequency (RF) spectroscopy. The LDOS is calculated as , where is the eigenvector corresponding to the eigenenergy ε n of Hamiltonian equation (4) and ν runs over all the Wannier orbitals ( s , p x or p y ) on A and B sites. We find that these gapless modes manifest themselves by a peak in LDOS located at the position of the domain wall, as shown in Fig. 2c–e . The reason for that peak of LDOS is the existence of localized gapless surface states, reminiscent of the quantum Hall edge states. This spatially localized zero-energy peak in LDOS can be detected using spatially resolved RF spectroscopy technique [39] . Taking a laser wavelength of λ =1,024 nm typical for the current optical lattices, the width of the LDOS peak is estimated about 2 μm. This is greater than the reported spatial resolution (about 1.4 μm) in the current experimental RF measurement [39] , which makes the detection of this signal experimentally accessible. Besides detecting edge properties, the bulk Chern number can also be used to demonstrate the topological nature of our proposed chiral p -wave superfluidity. For the detection of Chern numbers, one may adopt the existing proposals either from time-of-flight measurement [40] , [41] , [42] , [43] or from Bloch oscillation technique [44] , [45] . We now discuss the sharp distinction between our proposal to realize chiral p -wave superfluidity and that in previous studies [10] , [11] , [12] , [13] , [14] , [15] , [16] , [17] , [18] . Our proposed chiral p -wave superfluid state is a centre-of-mass p -wave superconducting pairing state. That is fundamentally different from other conventional p -wave superfluidity in previous studies, where the pairing order parameter has p -wave symmetry in the relative motion. The conceptual difference leads to two major distinct features in centre-of-mass p -wave state. One is that our proposal requires neither spin-orbit coupling nor an induced second-order effective p -wave interaction, automatically avoiding the challenge of their experimental realization in atomic Fermi gases. The centre-of-mass p -wave superfluidity proposed here arises directly from a purely s -wave two-body interaction. Hence, a short-ranged contact interaction as widely implemented in cold gases should satisfy well. This also significantly improves the transition temperature. The other feature is that the centre-of-mass p -wave superfluidity predicted here exhibits some unbroken symmetries such as spin U (1) symmetry and space lattice rotation symmetry. Such symmetries are absent in the conventional relative p -wave pairing state (for example, in spin-orbit-coupled fermion systems). We would like to stress that although the spin dependence of the studied lattice potentials is important to support our p -wave superconductivity in the weak interaction region, such lattices potentially causing experimental challenges could be avoided by considering strong interactions such as the resonance (see in Methods). The key ingredient for topological properties to emerge is rather from mixing Wannier orbitals of opposite parities. The connection between topological superconductivity and insulating or semimetalic phases [46] , [47] involving the idea of mixing parities remains an intriguing question for future research. In summary, we find a topological p -wave superfluid state in a spin imbalanced atomic Fermi gas with an s -wave interaction. Its pairing symmetry and topological origin differ from the previously known superconducting or superfluid phases. The p -wave symmetry refers to the centre-of-mass motion, not to the relative motion as in the well-known 3 He superfluid. The appearance of chiral fermionic zero modes bounded to domain walls is predicted as a concrete experimental signature for this novel state. After the submission of this manuscript, we became aware of a related paper [48] which puts forward an idea of generating p -wave interaction on the optical lattice. Spin-dependent optical lattice Experimentally, one may consider the existing proposals for realizing spin-dependent optical lattices [24] , [25] . Alternatively, the recent progress in group-II (alkaline-earth-metal) atoms points to the possibility of achieving even greater tunability by using the ground 1 S 0 and long-lived metastable 3 P 0 atomic levels, taking advantage of the strong orbit dependence of AC Stark effect in such systems. This should in principle be able to make the lattices for different components being completely independent (so maximally spin-dependent lattice) by selection of the appropriate wavelengths [25] . To be more specific, for the model presented here, we consider the lattice configurations for spin up ( s orbital) and down ( p orbital) fermions are V ↑ ( x , y )=− V s [cos 2 ( k ( x + y ))+cos 2 ( k ( x − y ))] and V ↓ ( x , y )=− V p [cos 2 ( kx )+cos 2 ( ky )], respectively. Here , V s and V p are the lattice strength, and λ is the wavelength of laser. The phase-stable lattices should in principle be realized through the phase control technique developed in recent experiments [49] , [50] . It is worthwhile to note that this special lattice configuration is to make the Cooper pair favourable even when interaction is weak. However, with strong interactions as in the resonance regime, such special lattice is expected to be unnecessary. The reason is that when the strong pairing-induced energy gap is a significant fraction of or is even comparable to the band width, Fermi surface nesting is no longer important for pairing. How to cite this article : Liu, B. et al. Chiral superfluidity with p -wave symmetry from an interacting s-wave atomic Fermi gas. Nat. Commun. 5:5064 doi: 10.1038/ncomms6064 (2014).